FoxP3+regulatory CD4 T cells control the generation of functional CD8 memory During the primary immune response, CD8 memory emerges from an environment of strong immune activation. The FoxP3 + regulatory CD4 T-cell subset (Treg) is known as a key suppressive component of the immune system. Here we report that Tregs are required for the generation of functional CD8 memory. In the absence of Tregs during priming, the resulting memory cells proliferate poorly and fail to differentiate into functional cytotoxic secondary effectors following antigen reactivation. We find that the Tregs act early, during the expansion phase of primary CD8 effectors, by fine tuning interleukin-2 exposure of CD8 memory precursors. This crucial new role of Tregs has implications for optimal vaccine development. On encountering antigens, naive CD8 T cells proliferate strongly and differentiate into primary effectors. This expansion step is followed by a phase of massive apoptosis ('contraction') in which only a minority of CD8 T cells survive to become highly competent memory cells [1] , [2] . Although CD4 T cells may not be essential for the generation of numerous primary CD8 effectors, particularly in inflammatory environments, lack of CD4 help during CD8 T-cell priming undermines the generation of CD8 memory [1] , [2] , [3] . Help from CD4 T cells also appears to be required for long-term memory CD8 T-cell maintenance [2] , [3] , [4] and reactivation on antigen re-exposure [5] , [6] , [7] , [8] , [9] , [10] . It is unclear whether different CD4 help signals are required for the different phases of CD8 memory responses, and whether they are provided by the same or distinct CD4 T-cell subsets. High levels of interleukin (IL)-2 or inflammatory cytokines, such as type I interferons and IFN-γ, may enhance CD8 T-cell expansion and differentiation into cytotoxic effectors but impair CD8 memory generation [11] , [12] , [13] , [14] . Conversely, low IL-2 signalling during the primary response may favour CD8 memory differentiation [12] , [13] , [14] . The level of IL-2 signalling can be controlled by regulation of CD25 (IL-2Rα) expression [12] , [14] , [15] . Upon its induction by TCR engagement, CD25 expression is under the control of IL-2 signalling and therefore relies on the availability of autocrine/paracrine IL-2 in the cell microenvironment [13] . Regulatory CD4 + CD25 hi FoxP3 T cells suppress immune responses and are important for peripheral immune tolerance [16] . Regulatory CD4 T cells (Tregs) rely on IL-2 of paracrine origin for their development, homoeostasis and suppressive functions, as they are unable to produce IL-2 themselves [16] . Strong CD25 expression on Tregs may therefore lead to competition for IL-2 secreted by activated CD4 and CD8 T cells. IL-2 consumption has been forwarded as a potential mechanism by which Tregs may regulate effector T-cell responses [17] , [18] , [19] . Here we examined the role of Tregs in the generation of CD8 memory. We found that Tregs control the level of IL-2 exposure of memory precursors during the primary immune response, enabling the development of functional CD8 memory. Tregs downregulate the expansion of CD8 T-cell effectors To examine the role of Tregs in the generation of CD8 memory following a primary CD8 T-cell response, we used FoxP3 + DTR mice, in which Tregs can be selectively and transiently depleted [20] . Mice were injected intravenously with 10 4 purified transgenic OT-I CD8 T cells. After 2 days, mice were immunized with OVA in complete Freund's adjuvant (CFA). After 3 days, they were treated with diphtheria toxin (DT) to deplete FoxP3 + CD4 T cells, which express CD25 ( Fig. 1a ). No significant Foxp3 expression was detected in total or OVA-specific CD8 T cells or in non-T cells, either in untreated mice or following OVA+CFA immunization ( Supplementary Fig. S1 ). The kinetics of Treg re-emergence following DT injection is shown in Fig. 1a . Treg depletion led to stronger expansion of OVA-specific CD8 primary effectors, which express a TCR specific for the immunodominant OVA 257–264 epitope (SIINFEKL) ( Fig. 1b,c ). This expansion was followed by contraction of the pool of primary effectors ( Fig. 1c ). However, at the end of the contraction process, the frequencies of OVA 257–264 -specific CD8 T cells remained higher than at baseline ( Fig. 1c ). Intriguingly, at the end of the primary effector contraction phase, the frequencies of OT-1 cells were similar whether or not DT was injected ( Fig. 1c ). Indeed, the amplitude of contraction was higher in Treg-depleted mice ( Fig. 1d ). This suggests that the amplitude of contraction may be proportional to the amplitude of expansion, regardless of the presence of Tregs, as these latter cells were still undetectable during the contraction phase in DT-treated mice ( Fig. 1a ). Alternatively, Tregs may specifically downregulate CD8 primary effector contraction, in which case the amplitude of contraction would be higher in their absence. To test this possibility, Tregs were depleted later, at the peak of effector expansion (days 5–6) ( Fig. 1c and Supplementary Fig. S2 ), just before the onset of contraction. This had no effect on the level of contraction ( Fig. 1d ). Thus, by contrast to their effect on the amplitude of CD8 effector expansion, Tregs appear to have no direct effect on the amplitude of contraction, which appears to depend rather on the amplitude of expansion. These results thus suggest that Tregs downregulate CD8 primary effector expansion. This was supported by the results of the in vitro experiments, in which Tregs and conventional CD4 T cells were cocultured with CD8 primary effectors. As shown in Fig. 2a , Tregs reduced the expansion of primary CD8 effectors. A point of particular interest is that neutralization of CD25 expressed by Tregs restored CD8 primary effector expansion ( Fig. 2a ). In the absence of Tregs, neutralization of CD25 expressed by CD8 T cells also reduced their expansion ( Fig. 2a ). We then used an IL-2 detection assay to examine the influence of Tregs on the level of IL-2 at the surface of CD8 T cells. As shown in Fig. 2b , Tregs reduced IL-2 availability at the surface of CD8 T cells, while CD25 neutralization on Tregs restored IL-2 levels at the surface of CD8 T cells. Together, these results suggest that Tregs, through their CD25 expression, downregulate the expansion of primary effector CD8 T cells, by competing for IL-2. 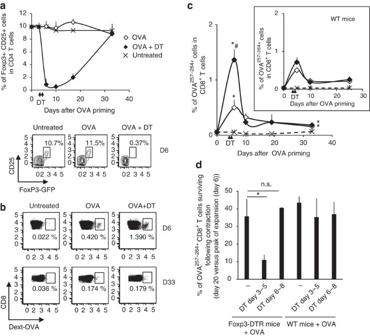Figure 1: Tregs control the amplitude of primary CD8 effector expansion. (a) FoxP3-DTR mice were injected with OT-I CD8 T cells and then vaccinated with OVA. On days 3 and 5, mice were injected with DT (OVA+DT) or not (OVA). The time course of the percentage of Foxp3+CD25+CD4+T cells after DT injection in untreated (crosses), OVA-treated (open diamonds) and OVA+DT-treated mice (closed diamonds) is shown. The arrows indicate DT injection on day 3 and day 5. A representative plot of FoxP3 and CD25 expression by CD4 T cells on day 6 is also shown. Panelbshows representative plots of OVA257–264-specific cell frequency in CD8+T cells on day 6 and day 33 in FoxP3-DTR mice treated as ina. (c) FoxP3-DTR mice and WT mice were injected with OT-I CD8 T cells then vaccinated with OVA. On days 3 and 5, mice were injected with DT (OVA+DT) or not (OVA). The time course of OVA257–264-specific CD8 T-cell frequency in Foxp3-DTR mice and WT mice (upper right graph) is shown. The arrows indicate DT injection on day 3 and day 5. *Significant versus untreated mice (P<0.01),#significant versus OVA-treated mice (P<0.01) (Wilcoxon test). (d) FoxP3-DTR mice and WT mice were injected with OT-I CD8 T cells then vaccinated with OVA. On days 3 and 5 or days 6 and 8, mice were injected with DT (OVA+DT) or not (OVA). The proportions of OVA257–264-specific CD8 T cells that survived following contraction (day 20 versus day 6 (peak of expansion)) are shown. Values were calculated as follows: 100−[100×(Fin treated mice−Fin untreated mice on day 20)/(Fin treated mice−Fin untreated mice on day 6)], whereFis the frequency of OVA257–264-specific CD8 T cells (*P<0.05, Wilcoxon test). The data ina,c,dare means±s.e.m. of six independent experiments with 2–3 mice per condition per experiment. Figure 1: Tregs control the amplitude of primary CD8 effector expansion. ( a ) FoxP3-DTR mice were injected with OT-I CD8 T cells and then vaccinated with OVA. On days 3 and 5, mice were injected with DT (OVA+DT) or not (OVA). The time course of the percentage of Foxp3 + CD25 + CD4 + T cells after DT injection in untreated (crosses), OVA-treated (open diamonds) and OVA+DT-treated mice (closed diamonds) is shown. The arrows indicate DT injection on day 3 and day 5. A representative plot of FoxP3 and CD25 expression by CD4 T cells on day 6 is also shown. Panel b shows representative plots of OVA 257–264 -specific cell frequency in CD8 + T cells on day 6 and day 33 in FoxP3-DTR mice treated as in a . ( c ) FoxP3-DTR mice and WT mice were injected with OT-I CD8 T cells then vaccinated with OVA. On days 3 and 5, mice were injected with DT (OVA+DT) or not (OVA). The time course of OVA 257–264 -specific CD8 T-cell frequency in Foxp3-DTR mice and WT mice (upper right graph) is shown. The arrows indicate DT injection on day 3 and day 5. *Significant versus untreated mice ( P <0.01), # significant versus OVA-treated mice ( P <0.01) (Wilcoxon test). ( d ) FoxP3-DTR mice and WT mice were injected with OT-I CD8 T cells then vaccinated with OVA. On days 3 and 5 or days 6 and 8, mice were injected with DT (OVA+DT) or not (OVA). The proportions of OVA 257–264 -specific CD8 T cells that survived following contraction (day 20 versus day 6 (peak of expansion)) are shown. Values were calculated as follows: 100−[100×( F in treated mice− F in untreated mice on day 20)/( F in treated mice− F in untreated mice on day 6)], where F is the frequency of OVA 257–264 -specific CD8 T cells (* P <0.05, Wilcoxon test). The data in a , c , d are means±s.e.m. of six independent experiments with 2–3 mice per condition per experiment. 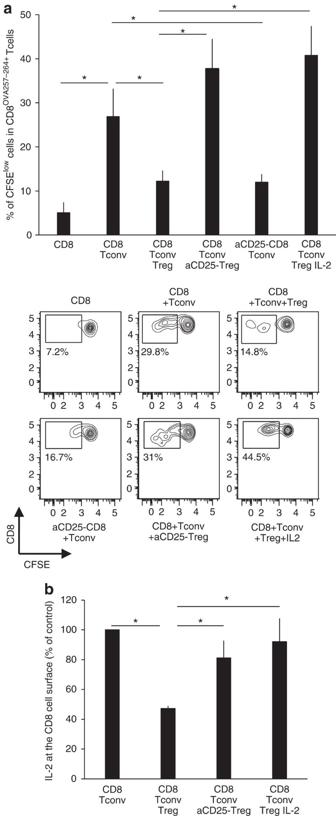Figure 2: Tregs reduce IL-2 exposure of CD8 T cells. (a) OT-I CD8 T cells were injected into WT mice before OVA vaccination. At 3 days after OVA vaccination, CD8 T cells were purified and labelled with CFSE. CD4 conventional cells (Tconv) and CD4 Tregs (Tregs) were purified from OT-II mice and preactivated separately for 3 daysin vitroby OVA-loaded mature DCs. Then CD4 and CD8 T cells were cocultured in the presence of OVA-loaded mature DCs. In some conditions, Tregs or CD8 T cells were preincubated in the presence of neutralizing anti-CD25 antibodies (aCD25-Tregs or aCD25-CD8). CFSE dilution was analysed in OVA257–264-specific CD8 T cells on day 3 of coculture. Results are expressed as the % of CFSElowcells and are the means±s.e.m. of four independent experiments performed in duplicate. Asterisks indicate statistically significant differences (P≤0.02, Wilcoxon test). Representative plot profiles are also shown. (b) CD4 and CD8 T cells were preactivated and cocultured as described ina, then IL-2 was detected at the surface of OVA257–264-specific CD8 T cells by using an IL-2 catch reagent (seeMethods). The results correspond to the % MFI versus control condition (CD8 T cells+CD4 Tconv coculture). Data are the means±s.e.m. of three independent experiments performed in duplicate. Asterisks indicate statistically significant differences (P<0.05, Wilcoxon test). Full size image Figure 2: Tregs reduce IL-2 exposure of CD8 T cells. ( a ) OT-I CD8 T cells were injected into WT mice before OVA vaccination. At 3 days after OVA vaccination, CD8 T cells were purified and labelled with CFSE. CD4 conventional cells (Tconv) and CD4 Tregs (Tregs) were purified from OT-II mice and preactivated separately for 3 days in vitro by OVA-loaded mature DCs. Then CD4 and CD8 T cells were cocultured in the presence of OVA-loaded mature DCs. In some conditions, Tregs or CD8 T cells were preincubated in the presence of neutralizing anti-CD25 antibodies (aCD25-Tregs or aCD25-CD8). CFSE dilution was analysed in OVA 257–264 -specific CD8 T cells on day 3 of coculture. Results are expressed as the % of CFSE low cells and are the means±s.e.m. of four independent experiments performed in duplicate. Asterisks indicate statistically significant differences ( P ≤0.02, Wilcoxon test). Representative plot profiles are also shown. ( b ) CD4 and CD8 T cells were preactivated and cocultured as described in a , then IL-2 was detected at the surface of OVA 257–264 -specific CD8 T cells by using an IL-2 catch reagent (see Methods ). The results correspond to the % MFI versus control condition (CD8 T cells+CD4 Tconv coculture). Data are the means±s.e.m. of three independent experiments performed in duplicate. Asterisks indicate statistically significant differences ( P <0.05, Wilcoxon test). Full size image Tregs control the development of functional CD8 memory We then examined whether the absence of Tregs during the primary CD8 T-cell response influences the generation of CD8 memory. The functionality of memory CD8 T cells that had developed in vivo in the presence or absence of Tregs was assessed in vitro following re-activation of splenocytes with OVA-loaded dendritic cells (DCs) for 4 days ( Fig. 3a ). This period of activation with DCs in the presence of CD4 T cells was necessary for secondary expansion of resting memory CD8 T cells and for their differentiation into cytotoxic secondary effectors [8] , [21] . As shown in Fig. 3b , stronger secondary expansion was observed when memory CD8 T cells had developed in the presence of Tregs. Similar results were observed for granzyme B secretion and cytotoxicity when re-activated memory OT-1 CD8 T cells were challenged with OVA-expressing target cells (E.G7-OVA cell line) ( Fig. 3c,d ). 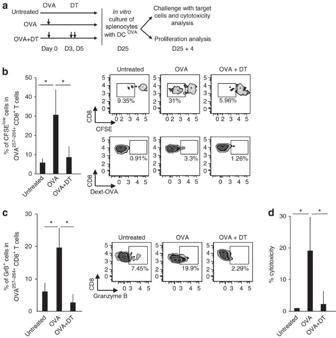Figure 3: Tregs favour the generation of functional CD8 memory followingin vitrochallenge. FoxP3-DTR mice were injected with OT-I CD8 T cells and then vaccinated with OVA. On days 3 and 5, they were either injected with DT (OVA+DT) or not injected (OVA). Splenocytes were isolated on day 25 and tested for proliferation, granzyme B production and cytotoxic activity (a). (b) Splenocytes were labelled with CFSE then cocultured for 4 days with OVA-loaded DCs. CFSE dilution was analysed in OVA257–264-specific CD8 T cells. Representative plots of CFSE dilution and frequencies of OVA257–264-specific cells in CD8 T cells are shown. (c) Splenocytes were cocultured with OVA-loaded DCs. After 4 days, OVA-expressing target cells (E.G7-OVA cell line, seeMethods) were added to the culture for 6 h. Granzyme B intracellular staining was performed in OVA257–264-specific CD8 T cells. Representative plots of Granzyme B staining of OVA257–264-specific CD8 T cells are shown. (d) Splenocytes were cocultured as inc. On day 4, CFSEloOVA target cells (E.G7-OVA cell line) and CSFEhicontrol cells (EL-4 cell line) were added to the culture. After 6 h, the CFSElo/CFSEhiratio was determined by flow cytometry. Percentage cytotoxicity was determined as described inMethods. Data are the means±s.e.m. of three independent experiments with 2–3 mice per condition per experiment. Asterisks indicate statistically significant differences (P<0.05, Wilcoxon test). Figure 3: Tregs favour the generation of functional CD8 memory following in vitro challenge. FoxP3-DTR mice were injected with OT-I CD8 T cells and then vaccinated with OVA. On days 3 and 5, they were either injected with DT (OVA+DT) or not injected (OVA). Splenocytes were isolated on day 25 and tested for proliferation, granzyme B production and cytotoxic activity ( a ). ( b ) Splenocytes were labelled with CFSE then cocultured for 4 days with OVA-loaded DCs. CFSE dilution was analysed in OVA 257–264 -specific CD8 T cells. Representative plots of CFSE dilution and frequencies of OVA 257–264 -specific cells in CD8 T cells are shown. ( c ) Splenocytes were cocultured with OVA-loaded DCs. After 4 days, OVA-expressing target cells (E.G7-OVA cell line, see Methods ) were added to the culture for 6 h. Granzyme B intracellular staining was performed in OVA 257–264 -specific CD8 T cells. Representative plots of Granzyme B staining of OVA 257–264 -specific CD8 T cells are shown. ( d ) Splenocytes were cocultured as in c . On day 4, CFSE lo OVA target cells (E.G7-OVA cell line) and CSFE hi control cells (EL-4 cell line) were added to the culture. After 6 h, the CFSE lo /CFSE hi ratio was determined by flow cytometry. Percentage cytotoxicity was determined as described in Methods . Data are the means±s.e.m. of three independent experiments with 2–3 mice per condition per experiment. Asterisks indicate statistically significant differences ( P <0.05, Wilcoxon test). Full size image We then examined the functionality of memory CD8 T cells in vivo 50 days after OVA priming, following in vivo reactivation of memory OT-1 CD8 T cells with injected OVA-loaded DCs ( Fig. 4a,b ) and subsequent in vivo challenge with OVA 257–264 peptide-loaded splenocytes ( Fig. 4a,c ). As shown in Fig. 4b,c , stronger secondary expansion and cytotoxicity were observed when memory CD8 T cells had developed in the presence of Tregs. Interestingly, Treg depletion at the peak of expansion, just before the onset of contraction, had no effect on CD8 T-cell memory, contrary to Treg depletion 3 days earlier ( Fig. 4b,c ), indicating that Tregs act mainly during the expansion phase of effector CD8 T cells. We also examined the functionality of CD8 memory generated in the presence and absence of Tregs after infection of mice with recombinant Listeria monocytogenes expressing the OVA fragment 134–387 (LmOVA) [22] , [23] , which includes the immunodominant OVA 257–264 epitope ( Fig. 4d ). As shown in Fig. 4e , control of bacterial replication was defective in mice in which OVA-specific CD8 memory had developed in the absence of Tregs. We then examined the control of bacterial replication on a per CD8 T-cell basis. The number of LmOVA CFU (colony-forming units) per 10 3 OVA 257–264 -specific CD8 T cells was 3,318±714 CFU in mice in which Tregs had been depleted during OVA priming, compared with only 62±28 in mice primed in normal conditions ( Fig. 4f ). Together, these results suggest that Tregs are required during CD8 primary effector expansion for the generation of highly functional CD8 memory. 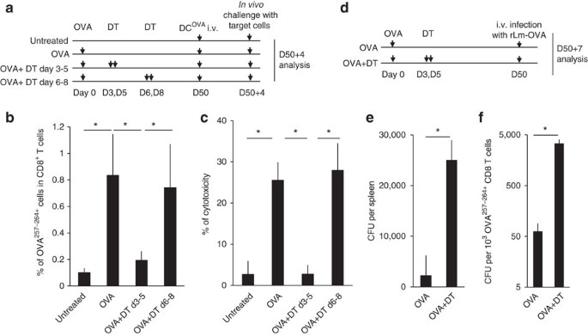Figure 4: Tregs favour the generation of functional CD8 memory following anin vivochallenge. (a) FoxP3-DTR mice were injected with OT-I CD8 T cells then vaccinated with OVA. Mice were injected with DT (OVA+DT) on days 3 and 5 or days 6 and 8, or not (OVA), and then, 50 days after priming, with OVA-loaded DCs. (b) Four days afterin vivoreactivation with OVA-loaded DCs, expansion of OVA257–264-specific CD8 T cells was analysed by flow cytometry. (c) Four days afterin vivoreactivation with OVA-loaded DCs, CFSE-labelled target cells were injected andin vivocytotoxic activity was determined 6 h later by analysing the CFSEhi/CFSElocell ratio among splenocytes, as described in Methods. Ind, 50 days after the priming, OVA- and OVA+DT-treated Foxp3-DTR mice were infected i.v. with 1.5×104CFU of rLm-OVA. The spleen bacterial load was determined 7 days later. Paneleshows the number of CFU per spleen in each condition. Panelfshows the number of CFU per 103OVA257–264-specific splenic CD8 T cells in each condition. Data are the means±s.e.m. of three independent experiments with 2–3 mice per condition per experiment. Asterisks indicate statistically significant differences (P<0.05, Wilcoxon test). Figure 4: Tregs favour the generation of functional CD8 memory following an in vivo challenge. ( a ) FoxP3-DTR mice were injected with OT-I CD8 T cells then vaccinated with OVA. Mice were injected with DT (OVA+DT) on days 3 and 5 or days 6 and 8, or not (OVA), and then, 50 days after priming, with OVA-loaded DCs. ( b ) Four days after in vivo reactivation with OVA-loaded DCs, expansion of OVA 257–264 -specific CD8 T cells was analysed by flow cytometry. ( c ) Four days after in vivo reactivation with OVA-loaded DCs, CFSE-labelled target cells were injected and in vivo cytotoxic activity was determined 6 h later by analysing the CFSE hi /CFSE lo cell ratio among splenocytes, as described in Methods. In d , 50 days after the priming, OVA- and OVA+DT-treated Foxp3-DTR mice were infected i.v. with 1.5×10 4 CFU of rLm-OVA. The spleen bacterial load was determined 7 days later. Panel e shows the number of CFU per spleen in each condition. Panel f shows the number of CFU per 10 3 OVA 257–264 -specific splenic CD8 T cells in each condition. Data are the means±s.e.m. of three independent experiments with 2–3 mice per condition per experiment. Asterisks indicate statistically significant differences ( P <0.05, Wilcoxon test). Full size image Memory CD8 T cells generated without Tregs overexpress PD-1 We then examined the in vivo expression of T-bet and TRAIL, two factors previously implicated in the defects of memory CD8 T cells generated in the absence of CD4 T cells [24] , [25] . T-bet has been reported to be overexpressed by helpless memory CD8 T cells [25] . As shown in Fig. 5a , T-bet expression by specific CD8 T cells increased during the primary response, in keeping with the role of T-bet in CD8 effector differentiation [26] . T-bet expression was higher in Treg-depleted mice but, following contraction, gradually fell to a level similar to that observed in CD8 T cells primed in the presence of Tregs ( Fig. 5a ). No clear expression of the pro-apoptotic factor TRAIL was found in specific CD8 T cells from either Treg-depleted or control mice during the 2 months following antigen priming ( Fig. 5b ), even after in vivo antigen reactivation with OVA-loaded DCs ( Fig. 5c ). In vivo expression of the inhibitory receptor PD-1 [27] was higher, for more than 1 month, in CD8 T cells primed in the absence of Tregs ( Fig. 5d ), subsequently falling to a level similar to that found in CD8 T cells primed in the presence of Tregs ( Fig. 5d ). However, following in vivo reactivation with OVA-loaded DCs, memory CD8 T cells generated in the absence of Tregs re-expressed higher levels of PD-1 ( Fig. 5e ). Strikingly, after in vivo infection with LmOVA, most OVA 257–264 -specific memory CD44 + CD8 T cells generated in the absence of Tregs expressed high levels of PD-1 ( Fig. 5f ). In addition, these cells did not upregulate the CD8 effector marker KLRG1 (killer cell lectin-like receptor G1) [28] , [29] , [30] , [31] , in keeping with the low granzyme B expression ( Fig. 5f and Supplementary Fig. S3a for KLRG-1 and Granzyme B expression in resting memory CD8 T cells). Therefore, CD8 secondary effectors derived from memory cells generated in the absence of Tregs had a KLRG − 1 − PD-1 high phenotype associated with severe functional impairment. 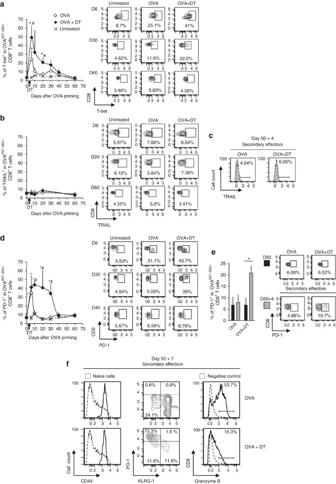Figure 5: Increased PD-1 expression in memory CD8 T cells generated in the absence of Tregs. FoxP3-DTR mice were injected with OT-I CD8 T cells then vaccinated with OVA. On days 3 and 5, mice were injected with DT (OVA+DT) or not (OVA). (a) Shows the time course of T-bet expression in OVA257–264-specific CD8 T cells for up to 60 days after priming (OVA-treated mice, open diamonds; OVA+DT-treated mice, closed diamonds; untreated mice, crosses). Representative plots are also shown. Positive cell gates were determined on the basis of isotype control staining. (b) Shows the time course of TRAIL expression in OVA257–264-specific CD8 T cells for up to 60 days after priming (OVA-treated mice, open diamonds; OVA+DT-treated mice, closed diamonds; untreated mice, crosses). Representative plots are also shown. (c) At 50 days after priming, OVA- and OVA+DT-treated mice received an injection of OVA-loaded DCs, and TRAIL was stained 4 days afterin vivoreactivation. Paneldshows the time course of PD-1 in OVA257–264-specific CD8 T cells for up to 60 days after priming (OVA-treated mice, open diamonds; OVA+DT-treated mice, closed diamonds; untreated mice, crosses). (e) At 50 days after priming, OVA- and OVA+DT-treated mice received an injection of OVA-loaded DCs, and PD-1 was stained 4 days after. (f) OVA or OVA+DT-treated FoxP3 DTR mice were challenged 50 days after priming with 1.5×104CFU of rLmOVA i.v. After 7 days, OVA257–264-specific CD8 T cells were analysed by flow cytometry for KLRG-1, PD-1, Granzyme B and CD44 expression. Results shown ina,b,dare the means±s.e.m. of 4–6 independent experiments with 2–3 mice per condition per experiment. Asterisks indicate statistically significant differences. *Significant versus untreated mice,#Significant versus OVA-treated mice (P<0.05 ina,P<0.02 ind, Wilcoxon test). Results shown inc,e,fare representative or the means±s.e.m. of 2–3 independent experiments with 2–3 mice per condition per experiment (*P=0.02, Wilcoxon test). Figure 5: Increased PD-1 expression in memory CD8 T cells generated in the absence of Tregs. FoxP3-DTR mice were injected with OT-I CD8 T cells then vaccinated with OVA. On days 3 and 5, mice were injected with DT (OVA+DT) or not (OVA). ( a ) Shows the time course of T-bet expression in OVA 257–264 -specific CD8 T cells for up to 60 days after priming (OVA-treated mice, open diamonds; OVA+DT-treated mice, closed diamonds; untreated mice, crosses). Representative plots are also shown. Positive cell gates were determined on the basis of isotype control staining. ( b ) Shows the time course of TRAIL expression in OVA 257–264 -specific CD8 T cells for up to 60 days after priming (OVA-treated mice, open diamonds; OVA+DT-treated mice, closed diamonds; untreated mice, crosses). Representative plots are also shown. ( c ) At 50 days after priming, OVA- and OVA+DT-treated mice received an injection of OVA-loaded DCs, and TRAIL was stained 4 days after in vivo reactivation. Panel d shows the time course of PD-1 in OVA 257–264 -specific CD8 T cells for up to 60 days after priming (OVA-treated mice, open diamonds; OVA+DT-treated mice, closed diamonds; untreated mice, crosses). ( e ) At 50 days after priming, OVA- and OVA+DT-treated mice received an injection of OVA-loaded DCs, and PD-1 was stained 4 days after. ( f ) OVA or OVA+DT-treated FoxP3 DTR mice were challenged 50 days after priming with 1.5×10 4 CFU of rLmOVA i.v. After 7 days, OVA 257–264 -specific CD8 T cells were analysed by flow cytometry for KLRG-1, PD-1, Granzyme B and CD44 expression. Results shown in a , b , d are the means±s.e.m. of 4–6 independent experiments with 2–3 mice per condition per experiment. Asterisks indicate statistically significant differences. *Significant versus untreated mice, # Significant versus OVA-treated mice ( P <0.05 in a , P <0.02 in d , Wilcoxon test). Results shown in c , e , f are representative or the means±s.e.m. of 2–3 independent experiments with 2–3 mice per condition per experiment (* P =0.02, Wilcoxon test). Full size image Tregs act by reducing IL-2 exposure of memory CD8 precursors As outlined above, Tregs may reduce IL-2 availability for effector CD8 T cells ( Fig. 2b ). We therefore examined whether IL-2 capture by Tregs during CD8 T-cell priming in vivo might contribute to their effect on CD8 memory. We first injected Tregs from wild-type (WT) mice into Treg-depleted FoxP3-DTR mice ( Fig. 6a ). This led to partial recovery of CD8 memory, possibly owing to the lower percentage of Tregs among CD4 T cells in reconstituted mice than in control (DT-untreated) FoxP3-DTR mice ( Fig. 6b–d ). We then selectively neutralized CD25 on Tregs before their injection to mice ( Fig. 6a ). This had no significant effect on Treg survival in vivo , as Tregs were detectable in the spleen 3 days later ( Fig. 6b ). However, CD25 neutralization abrogated the positive effect of Tregs on CD8 memory in vivo , in terms of secondary expansion, cytotoxicity and PD-1 expression ( Fig. 6c–e ). This suggested that Tregs promote the generation of functional CD8 memory through IL-2 capture. Interestingly, the absence of Tregs during CD8 T-cell priming led to impaired expression of Blimp-1 (a transcription factor associated with CD8 T-cell primary or secondary effector differentiation [30] , [32] , [33] ) on memory CD8 T cells following antigen reactivation ( Fig. 6f and Supplementary Fig. S3b for Blimp-1 expression in resting memory CD8 T cells). Similar defective Blimp-1 expression was observed when CD8 T cells were primed in the presence of Tregs treated with CD25-neutralizing antibodies ( Fig. 6f ). We then examined the effect of a direct reduction in IL-2 exposure of CD8 T cells. Injection of anti-CD25-treated CD8 T cells to Treg-depleted mice ( Fig. 7a ) led to generation of functional CD8 memory ( Fig. 7b ). Levels of Blimp-1 and PD-1 expression by secondary CD8 effectors were similar to those of CD8 memory cells generated in normal conditions ( Fig. 7b ). Together, these results suggest that Tregs, by regulating IL-2 exposure during CD8 T-cell priming, promote the generation of memory CD8 T cells capable of differentiating into functional secondary effectors. 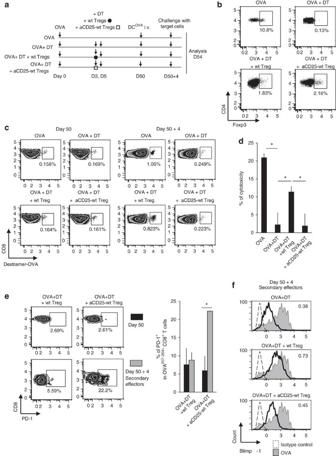Figure 6: Tregs favour the generation of functional CD8 memory through IL-2 capture. (a) FoxP3-DTR mice were injected with OT-I CD8 T cells and then vaccinated with OVA. On days 3 and 5, mice were injected with DT (OVA+DT) or not (OVA). Some OVA+DT-treated mice received an injection of either untreated Tregs (OVA+DT+Treg) or anti-CD25-preincubated Tregs (OVA+DT+aCD25 Treg) on day 3. Panelbshows the presence of injected Tregs on day 6. At 50 days after OVA priming, mice received an injection of OVA-loaded DCs (a). Panelcshows the frequency of OVA257–264-specific CD8 T cells in total CD8 T cells before (day 50) and after (day 50+4) 4 days ofin vivoreactivation by OVA-DCs. At 4 days after reactivation with OVA-loaded DCs, mice were injected with CFSE-labelled OVA-loaded splenocytes (a). (d)In vivocytotoxic activity was measured by flow cytometry 6 h later. In panele, PD-1 expression by OVA257–264-specific CD8 T cells was evaluated before and after 4 days of reactivation by OVA-DCs. A representative plot profile is also shown. In panelf, Blimp-1 expression by OVA257–264-specific CD8 T cells was analysed by flow cytometry after 4 days ofin vivoreactivation by OVA-DCs. Numbers in the top right corner represent the MFI ratio for each condition versus the OVA condition, calculated as follows: [(MFI sample−MFI isotype control)/(MFI OVA−MFI isotype control)]. Data inFigure 6are representative or the mean±s.e.m. of 2–3 independent experiments with 2–3 mice per condition per experiment. Asterisks indicate statistically significant differences (P≤0.02, Wilcoxon test). Figure 6: Tregs favour the generation of functional CD8 memory through IL-2 capture. ( a ) FoxP3-DTR mice were injected with OT-I CD8 T cells and then vaccinated with OVA. On days 3 and 5, mice were injected with DT (OVA+DT) or not (OVA). Some OVA+DT-treated mice received an injection of either untreated Tregs (OVA+DT+Treg) or anti-CD25-preincubated Tregs (OVA+DT+aCD25 Treg) on day 3. Panel b shows the presence of injected Tregs on day 6. At 50 days after OVA priming, mice received an injection of OVA-loaded DCs ( a ). Panel c shows the frequency of OVA 257–264 -specific CD8 T cells in total CD8 T cells before (day 50) and after (day 50+4) 4 days of in vivo reactivation by OVA-DCs. At 4 days after reactivation with OVA-loaded DCs, mice were injected with CFSE-labelled OVA-loaded splenocytes ( a ). ( d ) In vivo cytotoxic activity was measured by flow cytometry 6 h later. In panel e , PD-1 expression by OVA 257–264 -specific CD8 T cells was evaluated before and after 4 days of reactivation by OVA-DCs. A representative plot profile is also shown. In panel f , Blimp-1 expression by OVA 257–264 -specific CD8 T cells was analysed by flow cytometry after 4 days of in vivo reactivation by OVA-DCs. Numbers in the top right corner represent the MFI ratio for each condition versus the OVA condition, calculated as follows: [(MFI sample−MFI isotype control)/(MFI OVA−MFI isotype control)]. Data in Figure 6 are representative or the mean±s.e.m. of 2–3 independent experiments with 2–3 mice per condition per experiment. Asterisks indicate statistically significant differences ( P ≤0.02, Wilcoxon test). 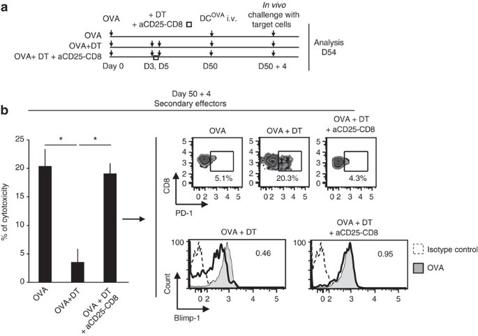Figure 7: Reduction of IL-2 exposure during priming restores the ability of CD8 T cells to generate functional memory cells. (a) FoxP3-DTR mice were injected with OT-I CD8 T cells and then vaccinated with OVA. On days 3 and 5, mice were either injected with DT (OVA+DT) or not injected (OVA). OVA+DT-treated mice received an injection of anti-CD25-preincubated CD8 T cells (OVA+DT+aCD25-CD8, seeMethods). At 50 days after OVA priming, mice received an injection of OVA-loaded DCs. After 4 days, mice were injected with CFSE-labelled OVA-loaded splenocytes. (b)In vivocytotoxic activity was measured by flow cytometry 6 h later. Representative plot profiles of PD-1 and Blimp-1 expression by OVA257–264-specific CD8 T cells are also shown. Numbers in the top right corner represent the MFI ratio for each condition versus the OVA condition, calculated as indicated in the legend to figure 6f. Data inFig. 7are the means±s.e.m. or representative of two independent experiments with 3 mice per condition per experiment. Asterisks indicate statistically significant differences (P<0.05, Wilcoxon test). Full size image Figure 7: Reduction of IL-2 exposure during priming restores the ability of CD8 T cells to generate functional memory cells. ( a ) FoxP3-DTR mice were injected with OT-I CD8 T cells and then vaccinated with OVA. On days 3 and 5, mice were either injected with DT (OVA+DT) or not injected (OVA). OVA+DT-treated mice received an injection of anti-CD25-preincubated CD8 T cells (OVA+DT+aCD25-CD8, see Methods ). At 50 days after OVA priming, mice received an injection of OVA-loaded DCs. After 4 days, mice were injected with CFSE-labelled OVA-loaded splenocytes. ( b ) In vivo cytotoxic activity was measured by flow cytometry 6 h later. Representative plot profiles of PD-1 and Blimp-1 expression by OVA 257–264 -specific CD8 T cells are also shown. Numbers in the top right corner represent the MFI ratio for each condition versus the OVA condition, calculated as indicated in the legend to figure 6f. Data in Fig. 7 are the means±s.e.m. or representative of two independent experiments with 3 mice per condition per experiment. Asterisks indicate statistically significant differences ( P <0.05, Wilcoxon test). Full size image Little information is available on the help provided by CD4 T-cell subsets during the different phases of the CD8 memory response. A critical aspect of CD4 help is its role during the priming phase of CD8 memory generation [1] , [2] , [3] . By using OVA in CFA immunization, we found that the Treg subset has a critical role during the expansion phase of primary CD8 effectors, enabling the development of functional memory CD8 T cells. This effect appears to be mediated by IL-2 capture by Tregs, through their constitutively high CD25 expression, which regulates IL-2 exposure of memory CD8 T-cell precursors. Exposure of CD8 memory precursors to high IL-2 levels therefore appears to hinder the generation of highly functional CD8 memory. Tregs had no direct influence on CD8 T-cell contraction, the amplitude of which was related to the amplitude of expansion. In addition, the frequency of specific memory CD8 T-cell precursors within the entire CD8 compartment following contraction was not affected by the presence or absence of Tregs during priming. This suggests that a constant population of memory precursors—cells programmed to survive the contraction phase—is generated during the amplification phase of the primary response, regardless of the presence of Tregs. However, in the absence of Tregs during priming, the resulting memory cells failed to differentiate into highly functional secondary effectors following antigen reactivation. This defect was associated with low expression of the transcriptional repressor Blimp-1, a key regulator of CD8 T-cell differentiation into cytolytic effector cells. Another key observation is the overexpression of the inhibitory receptor PD-1 following antigen reactivation. Generation of functional memory CD8 T cells therefore appears to result from the conjunction of two apparently independent phenomena during the primary response: first, the presence of memory precursors programmed to survive the contraction phase, and second, the regulatory effect of Tregs on IL-2 exposure of CD8 memory precursors. Tregs may either compete for IL-2 with all CD8 T cells present in their vicinity, which may include CD8 memory precursors and short-lived CD8 effectors, or interact preferentially with memory CD8 precursors. This putative targeting would imply that CD8 memory precursors express specific molecules allowing their recognition by Tregs. However, we found that the presence of Tregs was associated with a lower peak of primary effector expansion, suggesting that they compete for IL-2 with all CD8 T cells and not only with memory precursors, although we cannot rule out the possibility that a particular subset of Tregs might preferentially interact with CD8 memory precursors. The source of IL-2 available to CD8 T cells during the priming phase could be either autocrine [34] or paracrine [35] . Possible paracrine sources include activated effector CD4 T cells (the main IL-2 producer in vivo ) and DCs [36] . As both IL-2 provision by effector CD4 T cells [21] and IL-2 capture by Tregs may require close physical proximity [18] , generation of functional CD8 memory might involve the formation of cell–cell associations between several partners, including effector CD4 T cells, regulatory CD4 T cells and CD8 memory precursors. During these interactions, Tregs might fine tune the degree of IL-2 exposure of memory CD8 precursors, thereby favouring memory cell differentiation. Our results open the way for new investigations on the role of Tregs during primary immune response to pathogens. Indeed, through epigenetic changes, CD8 T-cell memory status corresponds to a state of high responsiveness to antigens that ensures better control of pathogen replication than that provided by primary effectors but could also have immunopathologic effects. Our finding that Tregs control the generation of CD8 memory suggests that the adaptive immune system has evolved to ensure that 'high-speed driving', represented by a highly functional CD8 memory response, cannot develop in the absence of an effective Treg braking system. Another possibility is that, during the primary response, the immune system may sense, through Tregs, the level of immune activation and therefore the potential for an immunopathologic reaction to a given antigen. When Tregs are overwhelmed by high IL-2 levels and cannot efficiently buffer IL-2 exposure of CD8 memory precursors, highly functional CD8 memory would be unable to develop. Together, these findings provide new insights into the mechanisms of CD8 T-cell memory generation. They reveal an unexpected facet of the immunosuppressive role of Tregs and may have important implications for the development of efficient vaccines. Mouse experiments All mice had the C57BL/6 background. WT C57BL/6 mice were purchased from Janvier (Le Genest-Saint-Isle), and OT-I and OT-II mice from Charles River Laboratories (L'Arbresles, France). FoxP3-DTR mice were kindly provided by Dr AY Rudensky (Memorial Sloan-Kettering Cancer Center, New York). These latter mice express the diphtheria toxin receptor (DTR) fused to enhanced green fluorescent protein under the control of the FoxP3 promoter. Their Tregs therefore selectively express DTR, allowing their depletion by DT exposure [20] . Mice were injected i.v. with 10 4 purified OT-I CD8 T cells to improve dextramer detection of OVA-specific cells, then vaccinated 2 days later (day 0) with 150 μg of purified OVA emulsified in CFA (Sigma-Aldrich). Some groups of mice received 500 ng of DT (Merck Chemicals) on days 3 and 5 after OVA+CFA vaccination to deplete Tregs at the start of detectable exposure to IL-2 and expansion of CD8 T cells (see Supplementary Fig. S2 ). Other groups of mice received DT on days 6 and 8, to deplete Tregs at the peak of expansion of CD8 primary effectors (see Supplementary Fig. S2 ). In some experiments, mice were injected with 500 OT-I CD8 T cells. This led to similar conclusions to those obtained with 10 4 injected OT-I cells (not shown). There was no need to distinguish between endogenous and adoptively transferred cells, as neither endogenous Foxp3-DTR CD8 T cells nor adoptively transferred TCR transgenic CD8 T cells express FoxP3, either at rest or following in vivo activation ( Supplementary Fig. S1 ). A recombinant strain of Listeria monocytogenes expressing the fragment 134–387 of OVA protein (rLM-OVA) was used for mouse challenge [22] . Mice were infected i.v. with 1.5×10 4 CFU of rLmOVA. After 7 days, the mice were killed, their spleens were removed and bacterial load was titrated by plating serial dilutions of spleen suspensions on BHI agar plates, as previously described [23] . The protocols were approved by the local ethics committee (Villejuif, France). Cells and culture The cell lines EL-4 and E.G7-OVA (a T-cell line expressing OVA peptides derived from EL-4 cells) were purchased from ATCC. DCs were isolated from the spleens of untreated WT mice (anti-CD11c microbeads, Miltenyi Biotec). Splenic DCs were loaded with OVA (2 μg ml −1 ) and matured with 0.5 μg ml −1 LPS (Sigma-Aldrich) for 24 h. CD8 T cells were isolated with magnetic beads (CD8α microbeads, Miltenyi Biotec). Conventional CD4 T cells (Tconv) and CD4 Tregs (Tregs) were purified from splenocyte populations by CD4-negative selection followed by CD25-positive selection (CD4 Treg isolation kit, Miltenyi Biotec). To analyse CD8 T-cell proliferation, splenocytes were stained with 0.5 μM CFSE. One million splenocytes were cocultured with 4×10 4 OVA-loaded DCs for 4 days. For Granzyme B analysis after CD8 T-cell reactivation, 10 5 E.G7-OVA cells per well were added to DC-splenocyte cocultures for 6 h in the presence of Brefeldin A (GolgiPlug, 1/1,000 v/v, BD Biosciences). For in vitro cytotoxicity assays after CD8 T-cell reactivation, E.G7-OVA cells were stained with 0.075 μM CFSE (CFSE lo ), and EL-4 cells were stained with 0.3 μM CFSE (CFSE hi ). The cells were then mixed at a 1/1 ratio, and 2×10 4 total cells per well were added to splenocyte-DC cocultures for 6 h. The cells were then analysed by flow cytometry and the CFSE lo /CFSE hi ratio ( R ) was determined in each condition. R control corresponds to CFSE lo /CFSE hi target cells incubated alone. Percentage cytotoxicity was determined as 100−( R ×100/ R control ). For OT-I/OT-II coculture, one WT mouse received purified OT-I CD8 T cells from one OT-I mouse and was then vaccinated with 150 μg of OVA protein emulsified in CFA. CD8 T cells were purified 3 days later. In parallel, purified CD4 Tconv and purified Tregs were isolated from OT-II mouse spleens and preactivated separately for 3 days with OVA-loaded mature DCs. Recombinant murine interleukin-2 (10 ng ml −1 , Immunotools) was added to Tregs. In some conditions, before coculture, Tregs or CD8 T cells were incubated for 2 h with anti-CD25 neutralizing antibodies (a mix of clones 3C7 and 7D4 from Southern Biotech Associates, each used at 15 μg ml −1 ). All cells were extensively washed. Then 5×10 5 CD8 T cells were cocultured for 3 days with 5×10 5 Tconv, 5×10 5 Tregs and 10 5 OVA-loaded DCs. In vivo transfer of Tregs or CD8 T cells Tregs from one WT mouse were purified (CD4 Treg isolation kit, Miltenyi Biotec), incubated for 2 h with anti-CD25 neutralizing antibodies (3C7 and 7D4, each at 15 μg ml −1 ) and washed extensively before i.v. injection. For CD8 T-cell transfer, a Foxp3-DTR mouse was injected i.v. with 10 4 purified OT-I CD8 T cells then vaccinated 2 days later (day 0) with 150 μg of purified OVA emulsified in CFA (Sigma-Aldrich). After 82 h later, total CD8 T cells were purified from the spleen, incubated for 2 h with anti-CD25 neutralizing antibodies (3C7 and 7D4, each at 15 μg ml −1 ) and washed extensively before i.v. injection. Antibodies and staining protocols The following reagents were used: anti-PD1-FITC or -PE-Cy7 (2 μg ml −1 ), anti-CD62L-FITC (0.5 μg ml −1 ), anti-CD8-FITC or -PE-Cy5 (1 μg ml −1 ), anti-CD44-PE (2 μg ml −1 ), anti-TRAIL-PE (2 μg ml −1 ), anti-T-bet-PE (2 μg ml −1 ), anti-Granzyme-B-PE (5 μg ml −1 ), anti-CD25-PE-Cy5 (2 μg ml −1 ), anti-Foxp3-APC (5 μg ml −1 ), anti-CD4-PE-Cy7 (0.5 μg ml −1 ) and anti-CD3-APC-Alexa750 (2 μg ml −1 ) (all from eBioscience), anti-KLRG-1-V450 (1 μg ml −1 ), anti-CD4-V500 (0.5 μg ml −1 ) (BD Biosciences), mouse dextramer-SIINFEKL-APC (5 μl per test, Immudex) and anti-BLIMP-1-PE (20 μl per test, Santa Cruz). Cells were acquired on a BD LSR Fortessa cytometer (BD Biosciences) and data were analysed with FlowJo software. For Foxp3 staining, cells were first stained with anti-CD4, -CD3, -CD8 and -CD25 antibodies, then fixed and permeabilized (FoxP3 Staining Set, eBioscience) and stained with anti-Foxp3-APC. For proliferation assays, CFSE-labelled cells were stained with dextramer SIINFEKL-APC followed by anti-CD3, -CD4 and -CD8 antibodies. CFSE dilution was analysed in the CD3 + CD4 − CD8 + dextramer-SIINFEKL + cell population. Results are expressed as the % of CFSE lo cells. For Granzyme B staining, cells were first stained with dextramer SIINFEKL-APC and anti-CD8/anti-CD4/anti-CD3 antibodies. The cells were then fixed and permeabilized (Cytofix/Cytoperm, BD Biosciences) then stained with anti-Granzyme-B-PE. For T-bet and BLIMP-1 staining, cells were first stained with dextramer SIINFEKL-APC and anti-CD8/anti-CD4/anti-CD3 antibodies, then fixed and permeabilized (FoxP3 Staining Set) and stained with either anti-T-bet-PE or anti-BLIMP-1-PE. Staining was analysed in the CD3 + CD4 − CD8 + dextramer-SIINFEKL + cell gate. For IL-2 catch assay, cells were labelled with IL-2 Catch Reagent according to the manufacturer's instructions (IL-2 secretion assay, Miltenyi Biotec), then incubated for 2 h at 37 °C before washing and staining with dextramer-SIINFEKL-APC, followed by anti-CD3, -CD4 and -CD8 antibodies. Captured IL-2 was then stained with anti-IL-2-PE (IL-2 secretion assay, Miltenyi Biotec) and surface-bound IL-2 was analysed in the CD3 + CD4 − CD8 + dextramer-SIINFEKL + cell gate. In vivo cytotoxicity assay Target cells were splenocytes coated with 10 μM class I-restricted peptide OVA 257–264 . Fifty days after priming, FoxP3-DTR mice were vaccinated i.v. with 10 6 OVA-loaded DCs. WT splenocytes were used as target cells. CFSE lo -labelled OVA 257–264 splenocytes (0.5 μM) and CFSE hi -labelled control splenocytes (5 μM) were mixed at a 1/1 ratio and 2×10 6 total cells were injected i.v. to FoxP3-DTR mice, 4 days after DC vaccination. The mice were killed 6 h later and the CFSE lo /CFSE hi ratio (termed R ) was determined in the live splenocyte gate. R control corresponded to the CFSE lo /CFSE hi target cell mix before injection to mice. Percentage cytotoxicity was determined as 100−( R ×100/ R control ). Statistical analysis The Wilcoxon test was used. How to cite this article: de Goër de Herve, M.G. et al . FoxP3 + regulatory CD4 T cells control the generation of functional CD8 memory. Nat. Commun. 3:986 doi: 10.1038/ncomms1992 (2012).